Josephson parametric phase-locked oscillator and its application to dispersive readout of superconducting qubits The parametric phase-locked oscillator (PPLO) is a class of frequency-conversion device, originally based on a nonlinear element such as a ferrite ring, that served as a fundamental logic element for digital computers more than 50 years ago. Although it has long since been overtaken by the transistor, there have been numerous efforts more recently to realize PPLOs in different physical systems such as optical photons, trapped atoms, and electromechanical resonators. This renewed interest is based not only on the fundamental physics of nonlinear systems, but also on the realization of new, high-performance computing devices with unprecedented capabilities. Here we realize a PPLO with Josephson-junction circuitry and operate it as a sensitive phase detector. Using a PPLO, we demonstrate the demodulation of a weak binary phase-shift keying microwave signal of the order of a femtowatt. We apply PPLO to dispersive readout of a superconducting qubit, and achieved high-fidelity, single-shot and non-destructive readout with Rabi-oscillation contrast exceeding 90%. The parametric phase-locked oscillator (PPLO) [1] , also known as a parametron [2] , is a resonant circuit in which one of the reactances is periodically modulated. It can detect, amplify, and store binary digital signals in the form of two distinct phases of self-oscillation. Indeed, digital computers using PPLOs based on a magnetic ferrite ring or a varactor diode as its fundamental logic element were successfully operated in 1950s and 1960s [2] . More recently, basic bit operations have been demonstrated in an electromechanical resonator [3] , and an Ising machine based on optical PPLOs has been proposed [4] . PPLOs also offer an interesting system to study fundamental physics of nonlinear oscillators [5] . Here using a PPLO realized with Josephson-junction circuitry, we demonstrate the demodulation of a microwave signal digitally modulated by binary phase-shift keying (BPSK). Moreover, we apply this demodulation capability to the dispersive readout of a superconducting qubit. This readout scheme enables a fast and latching-type readout, yet requires only a small number of readout photons in the resonator to which the qubit is coupled, thus featuring the combined advantages of several disparate schemes [6] , [7] . We have achieved high-fidelity, single-shot and non-destructive qubit readout with Rabi-oscillation contrast exceeding 90%, limited primarily by the qubit’s energy relaxation. PPLO with Josephson-junction circuitry Our PPLO is implemented by a superconducting coplanar waveguide (CPW) resonator defined by a coupling capacitor and a dc-SQUID (superconducting quantum interference device) termination ( Fig. 1a ; see Supplementary Fig. 1 and Supplementary Note 1 for the details of the device). The dc-SQUID, working as a controllable inductor, makes the resonant frequency of the resonator dependent on an external magnetic flux through the SQUID loop Φ sq (ref. 8 ). The application of a microwave field at a frequency ω p and a power P p to the pump line, which is inductively coupled to the SQUID loop, modulates the resonant frequency around its static value. This device has previously been operated as a Jopsehson parametric amplifier [9] , [10] . The signal at entering the resonator obtains a parametric gain produced by the pump at and is reflected back along the signal line. This device also works as a parametric oscillator when it is operated at P p above the threshold P p0 determined by the photon decay rate of the resonator [11] , [12] . Namely, it generates an output microwave field at ω p /2 even without any signal injection. The output can be one of the two degenerate oscillatory states (0 π and 1 π states) that differ solely by a relative phase shift π . 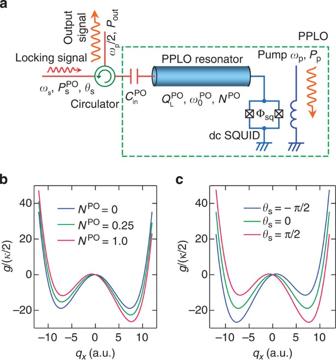Figure 1: Parametric phase-locked oscillator (PPLO). (a) Schematic of the device. The application of a pump microwave field atwith a powerPpabove the threshold generates an output signal atωp/2 with a powerPout. Here,is the static resonant frequency of the PPLO resonator, andωs,andθsrepresent the frequency, power and phase of the LS, respectively.represents the coupling capacitance between the resonator and the feedline, and Φsqrepresents the magnetic flux penetrating the SQUID loop. (b) Cross-section of the Hamiltoniang(qx, 0) in the rotating frame for various powers and a fixed phase (θs=π/2) of the LS. Here the LS power is represented by the mean photon number in the PPLO resonator,. Here the internal () and external () quality factors of the PPLO resonator are measured to be 5,200 and 340, respectively at, which give a loaded quality factorof 320. The pump powerPp/Pp0is fixed at 2.0. Two minima correspond to 0πand 1πstates of the phase-locked oscillations. (c) Same asb, but forNPO=1 and various values ofθs. Figure 1: Parametric phase-locked oscillator (PPLO). ( a ) Schematic of the device. The application of a pump microwave field at with a power P p above the threshold generates an output signal at ω p /2 with a power P out . Here, is the static resonant frequency of the PPLO resonator, and ω s , and θ s represent the frequency, power and phase of the LS, respectively. represents the coupling capacitance between the resonator and the feedline, and Φ sq represents the magnetic flux penetrating the SQUID loop. ( b ) Cross-section of the Hamiltonian g ( q x , 0) in the rotating frame for various powers and a fixed phase ( θ s = π /2) of the LS. Here the LS power is represented by the mean photon number in the PPLO resonator, . Here the internal ( ) and external ( ) quality factors of the PPLO resonator are measured to be 5,200 and 340, respectively at , which give a loaded quality factor of 320. The pump power P p / P p0 is fixed at 2.0. Two minima correspond to 0 π and 1 π states of the phase-locked oscillations. ( c ) Same as b , but for N PO =1 and various values of θ s . Full size image When an additional signal at ~ ω p /2 with a power , which we call the locking signal (LS), is injected into the parametric oscillator, the degeneracy of the two oscillatory states is lifted [13] . Such degeneracy lifting has been demonstrated in other physical systems such as magneto-optically trapped cold atoms [14] and electromechanical systems [15] . To understand the dynamics, we consider the Hamiltonian of the PPLO including a signal port for the LS and a fictitious loss port for internal loss of the resonator, namely, where γ represents the nonlinearity of the Josephson junction (JJ), a is the annihilation operator for the resonator, b k ( c k ) is the annihilation operator for the photon in the signal (loss) port with a wave number k and a velocity υ b ( υ c ), κ 1 ( κ 2 ) represents the coupling strength between the resonator and the signal (loss) port and κ = κ 1 + κ 2 . The equations of motion for the classical resonator field in a frame rotating at are obtained from the Hamiltonian by setting and are given by (ref. 16 ; also see Supplementary Note 2 for derivation) where and and θ s are the amplitude and phase of the LS, respectively. In the absence of the first term (oscillator’s friction term) on the right-hand side, equations (2) and (3) are in the form of Hamilton’s equations of motion with the Hamiltonian g ( q x , q y ), whose minima correspond to 0 π and 1 π states [16] . As shown in Fig. 1b , g ( q x , 0) is symmetric with respect to q x when there is no LS (| E s |=0), and 0 π and 1 π states are degenerate. When we apply LS, it gives a tilt to the double well, which is proportional to | E s | sin θ s ( Fig. 1b,c ). This lifts the degeneracy, and the PPLO, initially at q x , q y ~0, preferably evolves into one of the two states. This is how the amplitude and the phase of LS control the output state of the PPLO. Output of PPLO Now we show the experimental results. 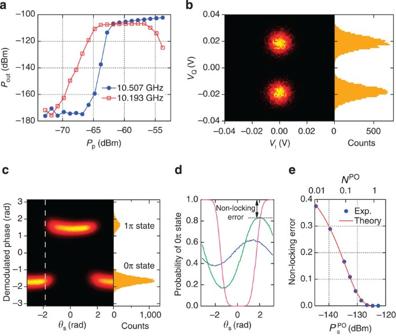Figure 2: Output of the PPLO. (a) Output signal power as a function ofPpat(solid blue circles) and(open red squares). The steep increase of the output power indicates onset of the parametric oscillation. Forb–e,is set to be 10.507 GHz. (b) Histogram of the amplitude and phase of the output signal plotted in the quadrature (IQ) plane (left panel) and its projection onto theVQaxis (right panel). The pulsed pump with a duration of 1.6 μs and an amplitude of −62 dBm is applied 1.6 × 104times in total. No LS is applied. (c) Histogram of the output-signal phase as a function of the LS phaseθs(left panel) and its cross-section along the dashed line (right panel). The same pulsed pump as inbis applied 2.0 × 104times for eachθs. LS is continuously applied with the power of −125 dBm. (d) Probability of 0πstate as a function ofθsforPsof −145 (blue), −135 (green) and −125 dBm (magenta). Phase shifts between different curves are an artefact due to the drift of the relative phase between the two generators used for the pump and the signal. In the qubit readout measurements, we used only one generator for the pump (with a frequency doubler) and the signal to avoid this problem. (e) Non-locking error as a function of the LS power. Solid blue circles represent the experimental data and the red curve is the result of a simulation based on the master equation. The corresponding mean photon number in the PPLO resonatorNPOis plotted on the top axis. Figure 2a shows the output power of the PPLO operated at (solid blue circles) as a function of P p in the absence of LS injection. For each P p , the microwave field is continuously applied to the pump port and the output signal at ω p /2 is measured by a spectrum analyser. Note that power levels stated in this work are referred to the corresponding ports on the chip. The steep increase of the output power at P p ~−65 dBm indicates the onset of the parametric oscillation. This is further confirmed by detecting the response to the pulsed pump. Figure 2b shows the histogram of the demodulated amplitude and phase of the output signal plotted in the quadrature (IQ) plane. For each application of the pump pulse with an amplitude of P p =−62 dBm, we recorded the output pulse and extracted its amplitude and phase by averaging for 100 ns. The two distribution peaks correspond to 0 π and 1 π states. They have equal amplitude but different phases shifted by π , and are observed with equal probabilities as expected. Figure 2: Output of the PPLO. ( a ) Output signal power as a function of P p at (solid blue circles) and (open red squares). The steep increase of the output power indicates onset of the parametric oscillation. For b – e , is set to be 10.507 GHz. ( b ) Histogram of the amplitude and phase of the output signal plotted in the quadrature (IQ) plane (left panel) and its projection onto the V Q axis (right panel). The pulsed pump with a duration of 1.6 μs and an amplitude of −62 dBm is applied 1.6 × 10 4 times in total. No LS is applied. ( c ) Histogram of the output-signal phase as a function of the LS phase θ s (left panel) and its cross-section along the dashed line (right panel). The same pulsed pump as in b is applied 2.0 × 10 4 times for each θ s . LS is continuously applied with the power of −125 dBm. ( d ) Probability of 0 π state as a function of θ s for P s of −145 (blue), −135 (green) and −125 dBm (magenta). Phase shifts between different curves are an artefact due to the drift of the relative phase between the two generators used for the pump and the signal. In the qubit readout measurements, we used only one generator for the pump (with a frequency doubler) and the signal to avoid this problem. ( e ) Non-locking error as a function of the LS power . Solid blue circles represent the experimental data and the red curve is the result of a simulation based on the master equation. The corresponding mean photon number in the PPLO resonator N PO is plotted on the top axis. Full size image Next we perform a similar measurement, but include LS injection. Figure 2c shows the histogram of the demodulated phase of the output signal as a function of the LS phase. While continuously injecting LS with a phase θ s and a power , we applied a pulsed pump with the same duration and the amplitude as in Fig. 2b , and extracted the phase of the output signal. As exemplified by the cross-section along the dashed line, the probabilities of obtaining the two states are no longer equal and depend on θ s . In Fig. 2d , we plot the probability of 0 π state as a function of θ s for different s. The probability shows sinusoidal dependence when is small. As we increase , the modulation amplitude (Δ P 0 π ) also increases and finally reaches unity. We define (1−Δ P 0 π )/2 as a non-locking error and plot it as a function of in Fig. 2e using blue circles. When is larger than ~−125 dBm (corresponding to N PO of 0.9), the non-locking error becomes negligible. We also simulated the non-locking error by solving a master equation [17] based on the Hamiltonian (equation (1)) and plot it by red curve (for details, see Supplementary Note 2 and Supplementary Figs 2 and 3 ). The only assumption here is the pump threshold P p0 , which is set to be −64.0 dBm. The agreement between the theory and the experiment is fairly good. Demodulation of BPSK signal The above result indicates the PPLO is a phase detector sensitive to very small microwave powers of the order of a femtowatt. To demonstrate this, we generate a signal digitally modulated by BPSK, a scheme commonly used in modern telecommunications [18] , and demodulate it by using a PPLO. 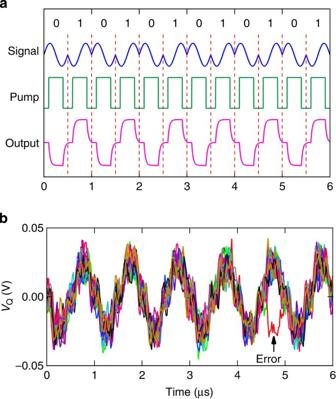Figure 3: Demodulation of BPSK signal. (a) Pulse sequence. BPSK signal at 10.503 GHz with an amplitude of −125 dBm is generated by mixing the 10.553 GHz signal and 50 MHz intermediate frequency (IF) signal (blue curve). Phase of the IF signal is digitally modulated byπ(corresponding to bit ‘0’ and bit ‘1’) every 500 ns and the pulsed pump (green curve) is synchronously applied. The magenta curve represents the expected output of the PPLO. (b) Examples of the demodulated signal. Twenty individual time traces are superposed. Figure 3a shows the sequence of the experiment. The generated signal has a fixed carrier frequency of 10.503 GHz, fixed power of −125 dBm and a phase that is digitally modulated by π every 500 ns. This means that the signal carries alternating binary bits with a baseband frequency of 2 MHz. Synchronously, we apply pump pulses with the duration of 300 ns and the amplitude of −62 dBm. Figure 3b shows the superposed time traces of the PPLO output. It shows successful demodulation of the input signal except rare errors as exemplified in the figure. We sent a total of 2.4 × 10 4 bits and detected four errors, corresponding to the error rate of 1.7 × 10 −4 . As studied in the parametron for its clock speed [19] , the response time of a PPLO decreases rapidly as we increase P p and . In the present study, we could make it comparable to the cavity decay time ( κ /2) −1 (see Supplementary Fig. 4 ). This time, together with the integration time to extract the output phase (100 ns in the present study), determines the upper limit for the baseband frequency of the BPSK signal to be demodulated, namely, the bandwidth of the PPLO as a phase detector. Figure 3: Demodulation of BPSK signal. ( a ) Pulse sequence. BPSK signal at 10.503 GHz with an amplitude of −125 dBm is generated by mixing the 10.553 GHz signal and 50 MHz intermediate frequency (IF) signal (blue curve). Phase of the IF signal is digitally modulated by π (corresponding to bit ‘0’ and bit ‘1’) every 500 ns and the pulsed pump (green curve) is synchronously applied. The magenta curve represents the expected output of the PPLO. ( b ) Examples of the demodulated signal. Twenty individual time traces are superposed. Full size image Qubit readout using PPLO Now we apply this phase discrimination capability to the dispersive readout of a qubit. 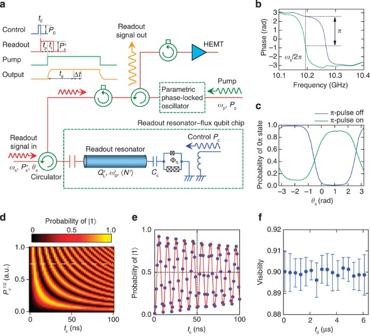Figure 4: Qubit readout using PPLO. (a) Measurement set-up and pulse sequence. A 3-JJ superconducting flux qubit biased at Φq=Φ0/2 is capacitively (Cc=4 fF) coupled to a CPW resonator. HereandNrrepresent the resonant frequency and the mean photon number of the readout resonator, respectively. The internal () and external () quality factors are 2.5 × 104and 630, respectively, resulting in the loaded quality factorof 620. In the pulse sequence, Δt(=100 ns) represents the data acquisition time to extract the phase, andandPcrepresent the power of the readout and the qubit control pulses, respectively. A short spike was added in the readout pulse to improve the readout fidelity. Inc–f, we applied the pulse sequence 1 × 104times to obtain the probability. (b) Frequency dependence of the phase of the reflection coefficient of the readout resonator with qubit controlπpulse on (green) and off (blue). (c) Probability of the PPLO 0πstate as a function of the readout-signal phaseθswith the qubit controlπpulse on (green) and off (blue). Heretc=10 ns,tp=50 ns,tr=50 ns andtd=300 ns. (d) Rabi oscillations measured withtp=30 ns,tr=50 ns andtd=300 ns. (e) Rabi oscillations along the dashed line ind. Red curve represents a fit with an exponentially damped sinusoidal function. (f) Visibility as a function oftd. Heretc=10 ns,tp=30 ns andtr=50 ns. The error bars represents the standard deviation in five identical measurements. Figure 4a shows the measurement set-up. A chip containing a 3-JJ superconducting flux qubit capacitively coupled to a CPW resonator (readout resonator) is connected to the PPLO via circulators. The flux qubit is biased at Φ q =0.5Φ 0 , where the qubit transition frequency from |0› to |1› states is 5.510 GHz. Figure 4b shows the phase rotation of the reflection coefficient around the resonant frequency of the readout resonator ( ) when the qubit is in |0› (blue) and |1› (green). The shift between the two curves is due to the dispersive coupling between the qubit and the readout resonator [20] . We set ω s to be 10.193 GHz, such that the qubit states are mapped onto two phases of the reflected microwave differing by π . Figure 4: Qubit readout using PPLO. ( a ) Measurement set-up and pulse sequence. A 3-JJ superconducting flux qubit biased at Φ q =Φ 0 /2 is capacitively ( C c =4 fF) coupled to a CPW resonator. Here and N r represent the resonant frequency and the mean photon number of the readout resonator, respectively. The internal ( ) and external ( ) quality factors are 2.5 × 10 4 and 630, respectively, resulting in the loaded quality factor of 620. In the pulse sequence, Δ t (=100 ns) represents the data acquisition time to extract the phase, and and P c represent the power of the readout and the qubit control pulses, respectively. A short spike was added in the readout pulse to improve the readout fidelity. In c – f , we applied the pulse sequence 1 × 10 4 times to obtain the probability. ( b ) Frequency dependence of the phase of the reflection coefficient of the readout resonator with qubit control π pulse on (green) and off (blue). ( c ) Probability of the PPLO 0 π state as a function of the readout-signal phase θ s with the qubit control π pulse on (green) and off (blue). Here t c =10 ns, t p =50 ns, t r =50 ns and t d =300 ns. ( d ) Rabi oscillations measured with t p =30 ns, t r =50 ns and t d =300 ns. ( e ) Rabi oscillations along the dashed line in d . Red curve represents a fit with an exponentially damped sinusoidal function. ( f ) Visibility as a function of t d . Here t c =10 ns, t p =30 ns and t r =50 ns. The error bars represents the standard deviation in five identical measurements. Full size image We discriminate the two states by using the PPLO and the pulse sequence shown in Fig. 4a . We set , ω p =2 ω s (corresponding to open red squares in Fig. 2a ) and P p =−65 dBm. Figure 4c shows the probability of detecting the 0 π state as a function of the phase of the readout microwave pulse θ s (similar to Fig. 2d ) with the qubit control π pulse off (blue) and on (green). The power of the readout microwave field at the input of the readout resonator is −120 dBm, which corresponds to the mean photon number in the readout resonator . Reflecting the π -phase difference of the reflected microwave field, the two curves are out of phase and their difference corresponds to the fidelity of the qubit readout, which is maximized at −2.0 and 1.2 rad to be 89%. We further maximized the fidelity by tuning t p and adding a short spike in the beginning of the readout pulse, and measured Rabi oscillations as shown in Fig. 4d , where the length t c and the amplitude of the qubit control pulse are swept. Figure 4e shows the Rabi-oscillation measurement along the dashed line in Fig. 4d . The contrast of the Rabi oscillations is 90.7%. We attribute the sources of the error to incomplete initialization of the qubit by 2.6% and to qubit energy relaxation (including the gate error of the π pulse), which adds 6.7%. Note that the non-zero minimum of the blue curve in Fig. 4c is due to incomplete initialization of the qubit and not the non-locking error. The non-locking error is confirmed to be negligible for both states of the qubit (see Supplementary Note 1 and Supplementary Figs 5 and 6 for the details). As stated above, N r of 5.5 is large enough to make the non-locking error of PPLO negligible. It is at the same time small enough for the qubit to avoid readout backaction. By sweeping t p , we can measure T 1 of the qubit, while populating photons in the readout resonator. It is measured to be 690 ns (see Supplementary Fig. 7 ), which agrees with T 1 obtained from the independent ensemble-averaged measurement using a standard pulse sequence, namely, a π pulse followed by delayed readout. This indicates the non-destructive character of the present readout scheme. Another characteristic of the present readout scheme is its latching property. Once the qubit state is mapped to the oscillator state of PPLO, the information can be maintained, regardless of a subsequent qubit state transition, as long as the pump is turned on. We demonstrate this in Fig. 4f , in which the readout fidelity is plotted as a function of t d . Even at t d =6 μs, at which the qubit has totally decayed, we do not lose readout fidelity. The present scheme enables fast, latching-type and single-shot readout of the qubit. In this sense, it is similar to schemes using a Josephson bifurcation amplifier [6] , Josephson-chirped amplifier [21] and period-doubling bifurcation [22] , where the qubit is directly coupled to a nonlinear resonator. However, in the present scheme, the mean photon number in the resonator to which the qubit is coupled can be kept small (of order unity) regardless of the result of the readout. In this sense, it is similar to schemes where a qubit is coupled to a linear resonator, followed by an ultra-low-noise amplifier such as Jopsehson parametric amplifier to achieve single-shot readout [10] . Thus, the present scheme has combined advantages of both linear and nonlinear resonators and can be useful in quantum error-correction protocols such as the surface code [23] . How to cite this article: Lin, Z. R. et al. Josephson parametric phase-locked oscillator and its application to dispersive readout of superconducting qubits. Nat. Commun. 5:4480 doi: 10.1038/ncomms5480 (2014).